Off-target-free gene delivery by affinity-purified receptor-targeted viral vectors We describe receptor-targeted adeno-associated viral (AAV) vectors that allow genetic modification of rare cell types ex vivo and in vivo while showing no detectable off-targeting. Displaying designed ankyrin repeat proteins (DARPins) on the viral capsid and carefully depleting DARPin-deficient particles, AAV vectors were made specific for Her2/neu, EpCAM or CD4. A single intravenous administration of vector targeted to the tumour antigen Her2/neu was sufficient to track 75% of all tumour sites and to extend survival longer than the cytostatic antibody Herceptin. CD4-targeted AAVs hit human CD4-positive cells present in spleen of a humanized mouse model, while CD8-positive cells as well as liver or other off-target organs remained unmodified. Mimicking conditions of circulating tumour cells, EpCAM-AAV detected single tumour cells in human blood opening the avenue for tumour stem cell tracking. Thus, the approach developed here delivers genes to target cell types of choice with antibody-like specificity. Specific detection, genetic modification and elimination of rare cell populations, such as micrometastases or circulating tumour cells (CTCs), are key challenges in cancer research, diagnostics and therapy. Of the tools to be developed for this purpose, in particular, gene transfer vectors derived from adeno-associated virus (AAV) have achieved broad attention due to the first granted marketing authorization for a gene transfer vector in the Western world [1] . As of yet, AAV is the vector of choice for in vivo gene function studies, owing to its excellent safety record and system-related features such as production at very high titres, low immunogenicity and efficient penetration through various types of tissue [2] . However, AAV vectors do show by nature a broad tropism, which results in transduction and loss of vector particles to irrelevant cells [1] (further on termed ‘off-targeting’). Attempts to tackle this challenge either focused on restricting transgene expression through tissue-specific promoters and/or post-translational targeting strategies [3] leaving the problem of off-target delivery untouched or on altering AAVs’ cell entry features by modifying the viral capsid. The latter approaches, referred here as cell entry targeting, either use adaptors possibly shielding the viral capsid from natural receptor binding and bridging between viral capsid and the chosen target receptor (non-genetic approaches) or permanently change the capsid by genetic engineering [4] , [5] . As of yet, genetic engineering employing DNA shuffling of capsid-encoding genes from different serotypes and directed evolution as means to select mosaic AAV capsids with novel features has demonstrated its promise as powerful strategy to improve, but not to restrict, gene delivery to a tissue of choice [5] , [6] , [7] . Similarly, efforts to redirect tropism by insertion of receptor-targeting peptides or by non-genetic targeting approaches were successful, but have so far not resulted in AAVs that do discriminate between defined cell types as specifically as, for example, antibodies or antibody mimetics can do [4] , [8] , [9] , [10] . Reasoning that specificity for a target receptor, and thus for a cell type of choice, is best achieved by displaying a high-affinity targeting domain based on a robust and well-folding scaffold, we recently exploited DARPins as targeting ligands [11] . Such target receptor-specific DARPins with affinities similar or better than those of antibodies can be obtained from libraries by selection approaches against essentially any molecule [12] and fold correctly even in the context of being fused to a virus capsid protein. For our proof-of-concept, we had employed a DARPin specific for Her2/neu [13] . Combining insertion of the Her2/neu-specific DARPin-9.29 as fusion to AAV’s capsid protein VP2 (viral protein 2) with ablation of natural receptor binding through mutagenesis of two arginine residues in each of the 60 capsid monomers resulted in an AAV vector preparation that was by far more specific for its target cells than any AAV vector developed so far [11] . However, a low, but detectable off-targeting in heart tissue remained. Hypothesizing that off-targeting is due to natural receptor-blinded AAV particles that lacked incorporation of the DARPin-VP2 fusion protein, we depleted our vector preparation for DARPin-deficient particles employing affinity chromatography. Through this additional step, we obtained Her2-AAV preparations that mediated target receptor-selective gene delivery, both ex vivo and in vivo , without any detectable off-target activity. Furthermore, we validated DARPin-deficient, natural receptor-blinded AAV particles as cause for the previously observed off-target activity and proved the flexibility and broad applicability of our strategy. In particular, we demonstrate reliable and precise transduction of micrometastases and CD4-positive T lymphocytes after systemic delivery of AAVs displaying DARPins specific for Her2/neu and for CD4, respectively. Moreover, AAVs targeted to EpCAM tracked rare tumour cells present in human blood with unprecedented efficiency. Separation of DARPin-displaying from DARPin-deficient AAV We recently reported on the development of a new AAV-targeting platform that exploited the N terminus of the viral capsid protein VP2 as insertion site for DARPin-based targeting ligands [11] . To redirect tropism, ligand insertion was combined with mutagenesis to eliminate key residues for natural receptor binding. VP2, however, is not essential for capsid assembly. Thus, viral vector preparations were expected to consist of both, DARPin-displaying and -deficient particles. The latter were assumed to be responsible for the off-targeting activity observed when administered in vivo . To separate DARPin-displaying from -deficient AAV particles, the DARPin-VP2 protein was His-tagged at the N terminus of the DARPin to allow immobilized metal ion affinity chromatography (IMAC) ( Fig. 1a , Supplementary Figs 1 and 2 ). When density gradient-purified Her2-AAV particles were loaded onto a HisTrap column, 16.6±6.1% of AAV particles were detectable in the flow-through and 68.6±10.2% ( N =3) in the elution fractions, resulting in a distinct peak ( Fig. 1b,c ; Supplementary Fig. 3a ). DARPin-displaying particles were only detected in the elution fractions ( Supplementary Fig. 3b ). More importantly, particles in the elution fraction were highly competent in transducing Her2/neu-positive SK-OV-3 cells, while particles present in the flow-through failed to do so ( Fig. 1d ). 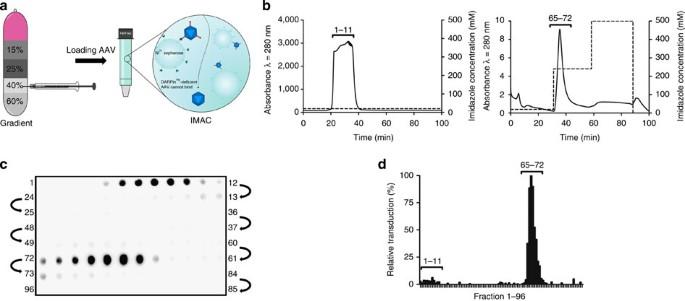Figure 1: Separation of DARPin-displaying from DARPin-deficient vector particles. (a) Schematic drawing of the two-step procedure including density gradient centrifugation followed by IMAC, which separates DARPin-displaying AAV particles carrying a hexa-histidine-tag at the N terminus of the DARPin from DARPin-deficient particles. (b) Example of chromatograms obtained after IMAC of a Her2-AAV vector stock. Left: Loading profile of iodixanol gradient-purified Her2-AAV vector preparations. Minutes 20–40 represent the loading of AAV particles, minutes 40–100 the column washing. Right: Elution profile of Her2-AAV particles. The absorbance at 280 nm is depicted. The loading and elution fraction numbers are indicated. The dashed line represents the imidazole concentration used during washing and elution. (c) 96 fractions collected during column loading (1–11), washing (13–49) and elution (65–72) were analysed by dot blot using the capsid protein-specific antibody B1. Fractions were loaded in alternating order from top left to bottom left as indicated by arrows. (d) Twenty μl of each fraction were used to transduce SK-OV-3 cells. The percentage of GFP-positive cells was quantified 60 h post transduction and is expressed relative to the highest transduction rate observed. Column loading and elution fractions are indicated. Figure 1: Separation of DARPin-displaying from DARPin-deficient vector particles. ( a ) Schematic drawing of the two-step procedure including density gradient centrifugation followed by IMAC, which separates DARPin-displaying AAV particles carrying a hexa-histidine-tag at the N terminus of the DARPin from DARPin-deficient particles. ( b ) Example of chromatograms obtained after IMAC of a Her2-AAV vector stock. Left: Loading profile of iodixanol gradient-purified Her2-AAV vector preparations. Minutes 20–40 represent the loading of AAV particles, minutes 40–100 the column washing. Right: Elution profile of Her2-AAV particles. The absorbance at 280 nm is depicted. The loading and elution fraction numbers are indicated. The dashed line represents the imidazole concentration used during washing and elution. ( c ) 96 fractions collected during column loading (1–11), washing (13–49) and elution (65–72) were analysed by dot blot using the capsid protein-specific antibody B1. Fractions were loaded in alternating order from top left to bottom left as indicated by arrows. ( d ) Twenty μl of each fraction were used to transduce SK-OV-3 cells. The percentage of GFP-positive cells was quantified 60 h post transduction and is expressed relative to the highest transduction rate observed. Column loading and elution fractions are indicated. Full size image We then analysed the biodistribution of particles from both fractions in comparison with particles not subjected to IMAC by injecting them into the tail vein of nude mice carrying a subcutaneously growing Her2/neu-positive tumour. We chose a vector dose for injection that was comparable to that administered in our previous study (2 × 10 10 vector genomes) (ref. 11 ). In all further in vivo experiments, the highest possible dose was administered, given the titre of each vector preparation. Vector stocks containing DARPin-displaying and -deficient particles resulted in on-target (tumour) and off-target (chest) transduction ( Fig. 2a ). Separating the two particle types by IMAC resulted in strong and exclusive luciferase activity in the tumour in those animals that had received the elution fraction (representing DARPin-displaying particles), while mice injected with the flow-through fraction showed strong signals in the chest region ( Fig. 2a ; Supplementary Fig. 4 ). 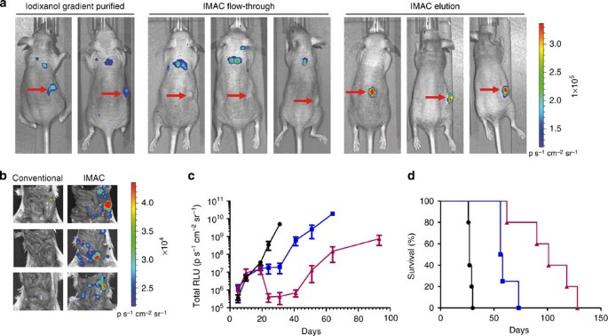Figure 2:In vivogene transfer by IMAC-purified Her2-AAV. (a) Her2-AAV encoding the luciferase gene was administered systemically into mice carrying subcutaneously growing SK-OV-3-derived tumours (arrow). Vector particles were administered intravenously by tail vein injection: iodixanol gradient-purified only (left;N=2), particles present in the flow-through (center;N=3), particles present in the elution peak fractions (right; N=3). Luciferase activity was monitored 1 week after vector administration. (b) Mice systemically injected with MDA-MB-453 cells received either IMAC-purified (right panels;N=3) or conventionally purified Her2-AAV (N=3) transferring the luciferase gene by tail vein injection. Images generated 7 days after vector administration show luciferase activities present in the gut expressed as photons/second/square centimetre/steradian (p s−1cm−2sr−1). (c) Mice that had been systemically injected on day 0 with luciferase-expressing MDA-MB-453-luc cells received a single intravenous injection of IMAC-purified HSV-TK-transferring Her2-AAV (5 × 1010vector genomes) on day 19, followed by GCV treatment for seven consecutive days (days 21–28; AAV group,N=5, purple triangles). The other groups received Herceptin according to established dosage regimes (days 21 and 27; Herceptin group,N=4, blue squares) or PBS only (mock group,N=5, black circles). The tumour burden was assessed regularly over 100 days byin vivoimaging and is expressed as relative light units (RLU), mean±s.e.m. Survival curves are shown ind. Statistics by Kaplan–Meier logrank test. Figure 2: In vivo gene transfer by IMAC-purified Her2-AAV. ( a ) Her2-AAV encoding the luciferase gene was administered systemically into mice carrying subcutaneously growing SK-OV-3-derived tumours (arrow). Vector particles were administered intravenously by tail vein injection: iodixanol gradient-purified only (left; N =2), particles present in the flow-through (center; N =3), particles present in the elution peak fractions (right; N=3). Luciferase activity was monitored 1 week after vector administration. ( b ) Mice systemically injected with MDA-MB-453 cells received either IMAC-purified (right panels; N =3) or conventionally purified Her2-AAV (N=3) transferring the luciferase gene by tail vein injection. Images generated 7 days after vector administration show luciferase activities present in the gut expressed as photons/second/square centimetre/steradian (p s −1 cm −2 sr −1 ). ( c ) Mice that had been systemically injected on day 0 with luciferase-expressing MDA-MB-453-luc cells received a single intravenous injection of IMAC-purified HSV-TK-transferring Her2-AAV (5 × 10 10 vector genomes) on day 19, followed by GCV treatment for seven consecutive days (days 21–28; AAV group, N =5, purple triangles). The other groups received Herceptin according to established dosage regimes (days 21 and 27; Herceptin group, N =4, blue squares) or PBS only (mock group, N =5, black circles). The tumour burden was assessed regularly over 100 days by in vivo imaging and is expressed as relative light units (RLU), mean±s.e.m. Survival curves are shown in d . Statistics by Kaplan–Meier logrank test. Full size image Elimination of disseminated tumour foci by Her2-AAV Notably, IMAC-purified Her2-AAV was not only more specific for its target cells but also more efficient in gene delivery than vector stocks containing both DARPin-displaying and -deficient particles. This was impressively demonstrated in a mouse model carrying widely disseminated Her2/neu-positive tumour cells present in various organs such as the gut and the lung. IMAC-purified Her2-AAV detected 75.7% (±10.6%; N =3) of the macroscopically visible tumour foci, while the non-IMAC-purified vector detected only 12.9% (±6.5%; N =3; Fig. 2b , Supplementary Fig. 5 ). To assess if delivery of an antitumoral gene will be therapeutically effective in this tumour model, we injected luciferase-labelled breast cancer-derived MDA-MB-453 cells into the tail vein. Once several sites of tumour growth were detectable by in vivo imaging, we started treatment with IMAC-purified Her2-AAV delivering the cytotoxic gene herpes simplex virus (HSV) thymidine kinase (TK), which converts ganciclovir (GCV) such that it becomes incorporated into DNA and stops replication. We compared this with the Her2/neu-specific monoclonal antibody Herceptin, an approved cancer drug, as control. Remarkably, a single injection of Her2-AAV followed by seven daily GCV administrations substantially reduced the tumour burden, before relapse occurred, while two administrations of Herceptin only halted tumour growth ( Fig. 2c ; Supplementary Fig. 6 , Supplementary Table 1 ), as expected from its well-described cytostatic action [14] . Consequently, Her2-AAV-treated mice survived significantly longer than Herceptin-treated mice ( Fig. 2d ). To demonstrate the flexibility of this targeting strategy, two further DARPins, previously described to bind to the surface receptors CD4 and EpCAM (epithelial cell adhesion molecule), respectively, were exploited as targeting ligands fused to the N terminus of VP2. Precise gene delivery to CD4-positive lymphocytes We chose CD4 as target aiming to generate a tool that specifically modifies CD4-positive immune cells that not only play a central role in protecting against infection and cancer, but are also the target of human immunodeficiency virus [15] . To specifically target this cell population, we decided to use DARPin 55_2, which performed best from a series of previously described human CD4-specific DARPins [16] . Like Her2-AAV, also CD4-AAV displaying the CD4-specific DARPin on its capsid surface readily discriminated between CD4-positive and CD4-negative lymphocyte cell lines ( Supplementary Figs 7 and 8 ). Moreover, IMAC-purified CD4-AAV was highly efficient in transducing primary human CD4-positive lymphocytes not only in cell culture ( Fig. 3a,b ), but also as a single low-dose systemic injection into mice transplanted with human peripheral blood mononuclear cells (PBMCs). In such mice, human lymphocytes mainly repopulate the spleen [17] . We observed strong luciferase activity in the spleen of mice injected with IMAC-purified CD4-AAV encoding this transgene, while CD4-AAV that was not affinity-purified—and thus contained both, DARPin-displaying and -deficient particles—resulted only in moderate signals in spleen and the chest region, as observed before for Her2-AAV ( Fig. 3c ). The on-target specificity of the signals was confirmed by depleting or enriching for human CD4-positive cells explanted from the spleen of the mice. Basically all of the luciferase gene copies present in spleen were detected in the CD4-enriched but not in the CD4-depleted cell fraction, resulting in transduction of 4.4±0.7% ( N =3) of all human CD4-positive spleen cells ( Supplementary Fig. 9 ), demonstrating clear evidence for the specific genetic modification of CD4-positive lymphocytes in vivo after systemic vector administration. 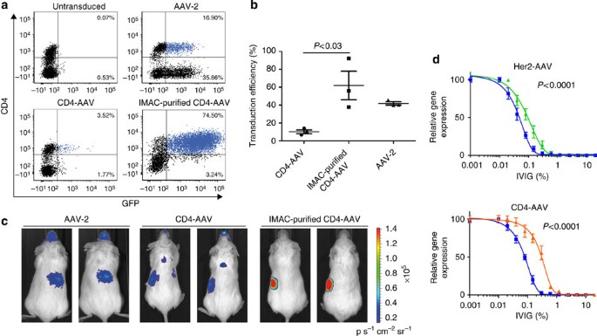Figure 3: Gene transfer into lymphocytes and sensitivity to human serum. (a) PBMCs were isolated, stimulated and transduced with either conventionally purified CD4-AAV (bottom left, 1.5 × 105vector genomes), IMAC-purified CD4-AAV (bottom right, 1.5 × 105vector genomes) or with AAV-2 (top right, 9 × 104vector genomes) or left untransduced (top left). Representative flow cytometry data are shown. (b) Statistical data ofa. Transduction efficiencies are expressed as percentage of GFP-positive cells.N=3, mean±s.d., statistics by two-tailedt-test. (c) NSG mice were systemically injected with stimulated human PBMCs. After 2 weeks, mice were injected with 5 × 109vector genomes of AAV-2 (left), conventionally purified CD4-AAV (center) or IMAC-purified CD4-AAV (right) vectors, respectively, transferring the luciferase gene. Luciferase activity was monitored on day 7 after vector administration. Luciferase signal intensity is expressed as photons/second/square centimetre/steradian (p s−1cm−2sr−1). Representative mice are shown.N=3. (d) CHO-Her2-k6 (top) or A3.01 (bottom) cells were transduced with equal amounts of Her2-AAV (green), CD4-AAV (orange) or AAV-2 (blue) vector particles encoding luciferase after incubation with serial dilutions of pooled human serum (IVIG) for 2 h at room temperature. After 72 h, cells were lysed and luciferase expression was analysed using the Dual-Luciferase Reporter Assay System (Promega). Data points were fitted using a non-linear regression;N=3 experiments; statistics by two-way analysis of variance; mean±s.d.;P<0.05 is considered to be statistically significant. Figure 3: Gene transfer into lymphocytes and sensitivity to human serum. ( a ) PBMCs were isolated, stimulated and transduced with either conventionally purified CD4-AAV (bottom left, 1.5 × 10 5 vector genomes), IMAC-purified CD4-AAV (bottom right, 1.5 × 10 5 vector genomes) or with AAV-2 (top right, 9 × 10 4 vector genomes) or left untransduced (top left). Representative flow cytometry data are shown. ( b ) Statistical data of a . Transduction efficiencies are expressed as percentage of GFP-positive cells. N =3, mean±s.d., statistics by two-tailed t -test. ( c ) NSG mice were systemically injected with stimulated human PBMCs. After 2 weeks, mice were injected with 5 × 10 9 vector genomes of AAV-2 (left), conventionally purified CD4-AAV (center) or IMAC-purified CD4-AAV (right) vectors, respectively, transferring the luciferase gene. Luciferase activity was monitored on day 7 after vector administration. Luciferase signal intensity is expressed as photons/second/square centimetre/steradian (p s −1 cm −2 sr −1 ). Representative mice are shown. N =3. ( d ) CHO-Her2-k6 (top) or A3.01 (bottom) cells were transduced with equal amounts of Her2-AAV (green), CD4-AAV (orange) or AAV-2 (blue) vector particles encoding luciferase after incubation with serial dilutions of pooled human serum (IVIG) for 2 h at room temperature. After 72 h, cells were lysed and luciferase expression was analysed using the Dual-Luciferase Reporter Assay System (Promega). Data points were fitted using a non-linear regression; N =3 experiments; statistics by two-way analysis of variance; mean±s.d. ; P <0.05 is considered to be statistically significant. Full size image Given the high prevalence for anti-AAV antibodies in the human population, a general concern with systemic administrations of AAV vectors refers to neutralizing antibodies that may substantially reduce gene delivery [5] . We therefore performed transduction experiments with Her2-AAV and CD4-AAV in the presence of pooled human serum (IVIG). Interestingly, we observed for both receptor-targeted AAVs an enhanced resistance towards neutralizing antibodies as compared with the parental AAV-2 ( Fig. 3d ). EpCAM-AAV detects tumour cells in human blood Epithelial cell adhesion molecule (EpCAM or CD326) was chosen due to its presence on human epithelial tissue and derived cancer cells [18] . Furthermore, EpCAM is described as surface marker of CTC, present in only low numbers in the blood of many cancer patients but equipped with strong invading and metastasizing potential [19] . Also the EpCAM-specific DARPin Ec1 (ref. 20 ) was efficiently displayed on the particle surface ( Supplementary Fig. 7 ) and mediated EpCAM-specific gene transfer, which was further enhanced by IMAC purification ( Supplementary Figs 10 and 11 ). Target cell specificity was further confirmed by specifically inhibiting gene transfer with the extracellular domain of EpCAM ( Supplementary Fig. 12b ). To assess the potency of EpCAM-AAV in detecting rare EpCAM-positive tumour cells, we then mixed low amounts of EpCAM-positive MDA-MB-453 tumour cells with isolated human PBMCs. EpCAM-AAV tracked basically all of the tumour cells, even when they only accounted for 0.3% of the cell mixture. The fluorescence intensity of these cells was at least 100-fold above that of EpCAM-negative cells ( Supplementary Fig. 13 ). This encouraging result prompted us to assess the transduction of tumour cells mixed into whole human blood ( Fig. 4a ). EpCAM-AAV detected more than 90% of tumour cells (constituting between several thousand down to a few hundred cells) present in several million blood cells ( Fig. 4b ). Remarkably, also when fewer than 100 tumour cells were present, most of these were tracked by EpCAM-AAV ( Fig. 4c ). Interestingly, EpCAM-AAV did not transduce any cell in tumour cell-free samples, suggesting that this approach may be less prone to false-positive signals than available detection systems that rely on antibodies ( Fig. 4c ). 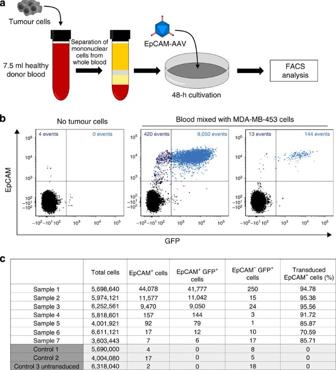Figure 4: EpCAM-AAV detects minimal numbers of tumour cells in human blood. (a) Workflow of the experimental procedure. Varying numbers of MDA-MB-453 tumour cells were mixed with 7.5 ml whole human donor blood and mononuclear cells were separated via density gradient centrifugation. The cell mixture was then transduced with EpCAM-AAV coding for GFP, cultivated for 48 h and analysed by flow cytometry for EpCAM and GFP expression. (b) Fluorescence-activated cell sorting (FACS) data of a sample containing whole blood without addition of MDA-MB-453 cells (left) or sample 3 (middle) and 4 (right) listed inc). Representative dot plots are shown. The number of events in each of the two gates containing EpCAM-positive cells is indicated. (c) Data overview for seven samples (samples 1–7) containing decreasing numbers of tumour cells and three controls (gray-shaded). Control 1 and 2 contained no tumour cells but were incubated with EpCAM-AAV, while control 3 contained neither tumour cells nor vector. Figure 4: EpCAM-AAV detects minimal numbers of tumour cells in human blood. ( a ) Workflow of the experimental procedure. Varying numbers of MDA-MB-453 tumour cells were mixed with 7.5 ml whole human donor blood and mononuclear cells were separated via density gradient centrifugation. The cell mixture was then transduced with EpCAM-AAV coding for GFP, cultivated for 48 h and analysed by flow cytometry for EpCAM and GFP expression. ( b ) Fluorescence-activated cell sorting (FACS) data of a sample containing whole blood without addition of MDA-MB-453 cells (left) or sample 3 (middle) and 4 (right) listed in c ). Representative dot plots are shown. The number of events in each of the two gates containing EpCAM-positive cells is indicated. ( c ) Data overview for seven samples (samples 1–7) containing decreasing numbers of tumour cells and three controls (gray-shaded). Control 1 and 2 contained no tumour cells but were incubated with EpCAM-AAV, while control 3 contained neither tumour cells nor vector. Full size image We present here the first gene delivery approach that achieved target specificity with antibody-like precision, both ex vivo and in vivo . In addition, it is highly modular and mediates efficient gene transfer, even if the target cell type is highly underrepresented or located in difficult to reach tissues such as a solid tumour. The flexibility of the system was confirmed by targeting different types of tumour cells and subtypes of lymphocytes. Despite capsid modifications, genomic titres of the DARPin-AAV preparations were comparable among each other ( Supplementary Fig. 14 ) and only marginally reduced compared with unmodified AAV vector particles. This is in line with our initial finding demonstrating that insertion of DARPins at the N terminus of VP2 does not interfere with capsid assembly or packaging efficiency [11] . DARPins are thus a further example proving the suitability of this insertion site for the display of functionally active polypeptides while keeping basic viral vector functions active [21] , [22] . After cell entry, Her2-AAV showed an overall similar intracellular distribution as the unmodified vector, AAV-2, with a small shift from nuclear to membrane-bound localization ( Supplementary Fig. 15 ). The kinetics of luciferase expression were significantly retarded for Her2-AAV and CD4-AAV, compared with AAV-2 ( Supplementary Fig. 16 ). While the data may hint to a reduced particle release from endosomes they further prove that the target cell specificity we observed was not influenced by alterations in post-entry steps. To modify AAV’s tropism on the cell entry level, two different approaches were previously used: (i) generation of AAV variants composed of shuffled capsid proteins and (ii) employing targeting ligands in non-genetic or genetic capsid engineering approaches. AAV variants have thereby been obtained which, for example, better penetrate the vitreous humor to reach the retina [7] , or exhibit improved transduction of human hepatocytes [6] or keratinocytes [23] . However, libraries consisting of shuffled capsids typically expand, but do not redirect viral tropism and, in addition, do not allow directing the selection towards a particular chosen receptor. Similarly, insertion of peptides into the viral capsid as well as equipping AAV vectors non-genetically with targeting ligands without destruction or shielding of the natural receptor binding sites will result in an expanded tropism [4] , [24] . With regard to genetic targeting approaches candidate peptides are commonly selected from phage or AAV peptide display libraries, which—due to technical constraints—contain only short peptides [8] , [9] , [10] , [23] , [25] . These are unlikely to reach binding affinities comparable to antibodies, because of the entropy loss when a small peptide is bound. To generate high-affinity and high-specificity interactions with receptors a stably folded domain is required as targeting ligand. The DARPin scaffold [26] was previously shown to be compatible with insertion at the N terminus of the viral capsid protein VP2, to fold well and to maintain its specificity [11] . Complete redirection of AAV’s tropism thus requires a natural receptor-‘blinded’ capsid as backbone, as we use here, combined with a complete depletion of targeting-domain-deficient particles. Using DARPins selected for binding to a given receptor [12] , [13] , [27] , a modular system has been engineered that allows for the first time precise targeting of AAV vectors in a predetermined way at the cellular and molecular level, while excluding gene transfer into irrelevant cells. Key to achieve receptor-specific gene delivery without detectable off-target transduction was the separation of DARPin-displaying particles from DARPin-deficient ones, which was possible by simple IMAC, exploiting the His-tag fused to the DARPin. AAV particles have been previously modified with His-tags to facilitate particle purification by HisTrap columns [28] , [29] . Moreover, position 587 of the AAV-2 capsid, previously identified as possible insertion site for His-tags [29] , has recently been exploited to separate DARPin-displaying and DARPin-deficient particles [30] . However, since His-tag and DARPin are not physically linked in this setting, recombination, which is a frequent event in packaging cells [31] , can give rise to DARPin-deficient but His-tag-displaying particles. Moreover, position 587 is embedded in the natural HSPG receptor binding motif [32] , [33] . The presence of positively charged residues as those of the His-tag at this position can reconstitute HSPG binding and natural receptor usage for cell entry [34] , [35] . Owing to these potential risks and the absence of a functional proof that a His-tag in position 587 indeed efficiently depletes DARPin-deficient particles [30] , we decided to place the His-tag N-terminally of the DARPin, thus avoiding both of the above mentioned risks. This step enhanced in addition gene delivery more than 10-fold. While the enhanced gene delivery to target cells can be expected from greatly enriching DARPin-displaying AAV particles ( Fig. 1b , left and right chromatogram), the reduced off-target transduction suggests that the presence of the DARPins interferes with the uptake of receptor-blinded vectors into non-target tissue. As an example, CD4-AAV, the as of yet first non-enveloped viral vector that efficiently transduces lymphocytes, modified CD4-positive human cells in the applied mouse model but did not detectably transduce any mouse or CD4-negative human cells. Moreover, Her2-AAV detected the majority of metastases present in a tumour mouse model after only a single systemic injection. Remarkably, this vector was more effective in reducing the tumour mass than Herceptin, a Her2/neu-specific therapeutic antibody currently in clinical use, albeit in combination therapy, for the treatment of breast cancer patients. Her2-AAV (delivering HSV-TK) was antitumorally effective already after a single intravenous administration followed by seven injections of GCV, before a relapse occurred. In contrast to Herceptin, effective cell killing can be exerted in absence of a fully functional immune system and chemotherapy, even though complete tumour elimination will require further optimizations. A general concern with systemic administrations of AAV vectors to patients refers to neutralizing antibodies that may substantially reduce gene delivery [5] . Interestingly, we observed an enhanced resistance towards neutralizing antibodies for receptor-targeted AAVs, suggesting that these vectors will be less sensitive towards inactivation by antibodies when administered to patients. Most likely, this is due to the mutations R585A and R588A, which were introduced to abolish natural receptor binding and are located near the highly immunogenic three-fold symmetry axis [36] . If required, this immune escape phenotype can be further improved by introducing additional mutations shown to interfere with binding of neutralizing antibodies [37] . Also, when administered to naïve patients, receptor-targeting may likely reduce the level of induced immune responses. Reasons are the potential reduction in vector dose required, and the restricted expression and thus presentation of transgene products in target cells. CTCs are a key cell type in today’s cancer diagnosis and for metastasis formation [38] . Detection of these cells is one of the main challenges in cancer prognosis. We show a proof of principle for EpCAM-AAV to specifically and efficiently detect tumour cells strongly underrepresented in human blood at a high signal-to-noise ratio. However, for an AAV-based CTC detection as a diagnostic tool, many parameters can still be further optimized. These include the use of single-stranded AAV vectors that may offer a second layer of specificity, as their need to undergo second strand synthesis before transgene expression is hampered in cells of the hematopoietic system, but proceeds efficiently in tumour cells [39] , [40] . Plasmids For the generation of plasmids encoding the DARPin-VP2 fusion constructs, the reading frames of the Her2-specific DARPin-9.29 (ref. 13 ), the CD4-specifc DARPin 55_2 (ref. 16 ) and the EpCAM-specific DARPin Ec1 (ref. 20 ) were amplified by PCR using the primer pair DARPin-for/DARPin-rev or DARPin-for/DARPin EC1-rev respectively, ( Supplementary Table 1 ) and were inserted into pGFP (green fluorescent protein)-VP2 (ref. 21 ) by sticky-end ligation using AgeI and BsrGI restriction sites resulting in plasmids pHer2-VP2, pCD4-VP2 and pEpCAM-VP2. Plasmids encoding VP2 fused to His-tagged or Myc-tagged DARPins were generated analogously using the primer pairs His-forw/DARPin-rev or His-forw/DARPin EC1-rev and Myc-forw/DARPin-rev or Myc-forw/DARPin Ec1-rev, respectively. All AAV vectors were of self-complementary conformation and encoded gfp (pscGFP; 2,200 base pairs including ITRs), GL4-luciferase (pscLUC; 3,100 base pairs including ITRs) or HSV-TK (pscHSV-TK; 2,600 base pairs including ITRs) [11] under control of the strong and ubiquitously active spleen focus-forming virus promoter [41] . Vector particle production AAV-targeting vectors and AAV-2 were generated using the adenovirus-helper-free AAV-packaging strategy [42] . HEK-293 cells (2.4 × 10 7 ) were seeded 24 h before transfection into 15 cm cell culture dishes and transfected using polyethyleneimine. Before transfection, the medium was replaced with 10 ml Dulbecco’s modified Eagle medium (DMEM) supplemented with 15% fetal calf serum (FCS) and 2 mM glutamine. In total, 11.25 μg of the helper plasmid pXX6-80 (ref. 42 ), 3.75 μg pRCVP2koA, 3.75 μg pDARPin-VP2 and 3.75 μg of the transfer vector plasmid were mixed with 2 ml DMEM. In parallel, 120 μl 18 mM polyethyleneimine and 2 ml DMEM were mixed. Both the solutions were combined and incubated for 20 min at room temperature (25 °C). After adding 1 ml DMEM supplemented with 2 mM glutamine, the mixture was added to the cells. Twenty-four hours later, the medium was replaced with 20 ml DMEM supplemented with 15% FCS and 2 mM glutamine. Forty-eight hours after transfection, cells were scraped off, pelleted (200 g , 7 min, 4 °C) and lysed using Tris-HCl NaCl, pH 8.5. After Benzonase (Sigma-Aldrich, Hamburg, Germany) treatment (50 U ml −1 cell lysate, 30 min, 37 °C), cleared lysates (3,700 g , 20 min, 4 °C) were purified by iodixanol gradient purification for 2 h at 290,000 g in a Beckman 70Ti rotor and harvested from the 40% iodixanol layer. Immobilized metal ion affinity chromatography IMAC of DARPin-displaying AAV vector particles was performed using HisTrap HP nickel columns (GE Healthcare, Munich, Germany) and a HPLC system (Knauer, Berlin, Germany). For analytical chromatography, 100 μl iodixanol gradient-purified AAV preparation were diluted in 300 μl binding buffer (20 mM imidazole, 20 mM sodium phosphate, 0.5 M NaCl, pH 7.4) and injected into the equilibrated HPLC system. After particle loading, columns were washed with 10 column volumes of binding buffer and vector particles were subsequently eluted in 0.3 ml fractions using five column volumes of elution buffer containing 240 or 300 mM imidazole. Collected fractions were subsequently analysed by dot blot analysis. For preparative vector particle purification, 1.5 ml AAV stock collected from the iodixanol gradient was diluted in 3 ml binding buffer and purified as described above. Peak fractions were pooled and dialysed two times against a 1,000-fold volume of PBS overnight at 4 °C. Mouse models For subcutaneous tumour models, 6- to 8-week-old female Beige nude mice (Harlan Laboratories, Eystrup, Germany) were subcutaneously injected with 5 × 10 6 SK-OV-3 cells in 100 μl PBS into the right flank and intravenously administered with 1.5 × 10 10 vector genomes (vg) of indicated AAV vector preparations by tail vein injection 14 days after engraftment. For in vivo imaging of the activity of the GL4-luciferase (Promega, Mannheim, Germany), mice were intraperitoneally injected with 150 mg D -luciferin per kg body weight (Caliper Life Sciences, Mainz, Germany) and anaesthetized by isoflurane inhalation. Imaging data were obtained 10 min after substrate injection using a noninvasive cooled charged-coupled device (IVIS Spectrum; Caliper Life Sciences). Data were analysed using the Living Image Software (Caliper Life Sciences). For the disseminated tumour models 6- to 8-week-old female NOD.Cg-Prkdc scid Il2rg tm1Wj l/SzJ (further on termed ‘NSG’) (The Jackson Laboratory, Bar Harbor, USA) mice were engrafted with 2 × 10 6 MDA-MB-453 cells by tail vein injection and received 1 × 10 10 vector genomes of indicated vector preparations 12 days after cell administration by intravenous tail vein injection. Tumour lesions were subsequently confirmed by an experienced pathologist. For tumour killing experiments, 6- to 8-week-old female NSG mice were engrafted with 2 × 10 6 luciferase-expressing MDA-MB-453-luc cells by intravenous tail vein injection. They received a single intravenous tail vein injection of 5 × 10 10 vg of HSV-TK-transferring IMAC-purified Her2-AAV on day 19 after cell injection. From day 21–28, mice received a daily intraperitoneal injection of GCV (Cymevene, Roche, Basel, Switzerland) (100 mg kg −1 body weight, in PBS) for seven consecutive days or were treated with either 5 mg kg −1 body weight Herceptin (Roche, Basel, Switzerland) or PBS on day 21 and 27. Tumour burden was monitored by in vivo imaging of the total body luciferase signal in regular intervals. For transplantation of human PBMCs, 6- to 8-week-old female NSG mice were used. PBMCs purified from a buffy coat were stimulated using 100 U ml −1 interleukin-2 and 5 μg ml −1 anti-CD28 and anti-CD3 (eBioscience, San Diego, USA) antibodies for 3 days and transplanted by intravenous tail vein injection (8 × 10 6 cells). After mice had reached a human CD45 level of 10–15% in blood, they received 5 × 10 9 vg of CD4-AAV coding for luciferase by injection into the tail vein. Luciferase expression was determined by in vivo imaging. All experimental mouse work was carried out in compliance with the German animal protection law as approved by the Regierungspräsidium Darmstadt, Germany. Neither samples nor animals were excluded from the study and sample analysis was blinded. Western blotting 2 × 10 10 vector genomes containing the DARPin-9.29-VP2 fusion protein, with the two point mutations R585A and R588A but no hexa-histidine motif and Her2-AAV His (2 × 10 10 vector genomes), additionally containing a hexa-histidine motif, were analysed on an 8% SDS-polyacrylamide gel. Proteins blotted on a nitrocellulose membrane (Amersham Biosciences, Freiburg, Germany) were detected using either the capsid protein-specific antibody B1 recognizing VP1, VP2 and VP3 because of their identical C-terminal region (Progen, Heidelberg, Germany) or a hexa-histidine motif-specific antibody (Cell Signaling, Danvers, US). Signals were visualized by enhanced chemiluminescence using the ECL Plus Western Blotting Detection System (GE Healthcare, Munich, Germany). Images have been cropped for presentation. Full-size images are presented in Supplementary Fig. 17 . Dot blot analysis Twenty-five μl (for the detection of capsid proteins) or 100 μl (for the detection of the hexa-histidine motif) of collected fractions were mixed with 1% SDS and incubated for 10 min at 95 °C. Samples were blotted onto nitrocellulose membranes (GE Healthcare, Munich, Germany) using a dot blot apparatus (BioRad, Hercules, USA). Membranes were blocked with blocking buffer (5% milk powder in TBS-T (10 mM Tris-HCl, 0.1% Tween 20, pH 8.0)) for 1 h at room temperature and incubated with either the capsid protein-specific antibody B1 (1:20 diluted) or with an anti-His mAb (1:1,000 diluted; Cell Signaling, Danvers, USA). Final detection was performed using HRP-conjugated rabbit anti-mouse immunoglobulins. Protein detection was performed using the Amersham ECL Plus western blotting detection reagent (GE Healthcare, Munich, Gemany). Enzyme-linked immunosorbent assay AAV fractions were coated on Maxisorp immunoplates (Nunc, Wiesbaden, Germany) and detected using the anti-AAV-2-capsid antibody A20 (1:4 diluted). Plates were incubated with a donkey anti-mouse biotin-conjugated antibody (Jackson Immuno Research, West Baltimore Pike, USA) (1:25,000 diluted) and HRP-conjugated streptavidin (1:500 diluted) (Dianova, Hamburg, Germany). Final detection was performed using TMB liquid substrate (Sigma-Aldrich, Hamburg, Germany). Analysis of mouse spleen Spleens were explanted and cell suspensions were prepared. CD4-positive cells were separated from CD4-negative cells using human anti-CD4 MicroBeads (Miltenyi Biotech, Bergisch Gladbach, Germany) and analysed for the amount of CD4-positive cells by flow cytometry and for the quantity of luciferase gene copies by qPCR using the primer pairs luc-for and luc-rev ( Supplementary Table 2 ). Competition assay CD4-AAV or EpCAM-AAV were incubated for 1 h at 4 °C with increasing amounts of the entire extracellular domain of human CD4 or human EpCAM (Sino Biological, Beijing, China). Following incubation, A3.01 or MDA-MB-453 cells were transduced and analysed for GFP expression by flow cytometry 72 h post transduction. Intracellular AAV distribution SK-OV-3 cells (1 × 10 6 ) were transduced with AAV-2 or Her2-AAV at a dose of 30,000 vector genomes per cell transferring the GFP gene. Cells were kept on ice for 45 min before incubation at 37 °C for 8 h. After harvesting of cells by trypsin treatment and subsequent washing in PBS, cell fractionation was performed (Subcellular protein fractionation kit, Thermo Scientific, Schwerte Germany). Cytoplasmic, membrane and nuclear fractions were collected and used in total for determining vector copy number per cell fraction. Specifically, DNA was isolated from the indicated fractions using DNeasy Blood and tissue kit (Qiagen, Hilden Germany) and was eluted in Tris/HCI. Vector copy numbers were quantified by LightCycler 480 qPCR (Roche, Basel Switzerland) using SYBR Green and transgene (GFP)-specific primers (eGFPfw, eGFPrev; Supplementary Table 2 ). Neutralization assay CHO-Her2-k6 or A3.01 cells were transduced with equal amounts of Her2-AAV, CD4-AAV or AAV-2 vector particles encoding luciferase after incubation with serial dilutions of IVIG (lntratect, Biotest, Dreieich, Germany) for 2 h at room temperature. After 72 h, cells were lysed and luciferase expression was analysed using the Dual-Luciferase Reporter Assay System (Promega, Mannheim, Germany). Detection of tumour cells in whole blood samples Blood (7.5 ml) of healthy donors was mixed with MDA-MB-453 cells and PBMCs were purified by density gradient centrifugation (30 min, 720 g ) using Histopaque (Sigma-Aldrich, Hamburg, Germany). Remaining erythrocytes were subsequently lysed (20 min, 37 °C, 0.86% ammonium chloride), washed with PBS and plated in a 10 cm 2 cell culture dish and 3 × 10 10 vg EpCAM-AAV were added. After 48 h, cells were completely removed from the cell culture dish using trypsin, washed, incubated with human FcR blocking reagent for 15 min on ice (20 μl per 10 7 cells, Miltenyi Biotec, Bergisch Gladbach, Germany) and stained with anti-CD326-PE (diluted 1:10, Miltenyi Biotec, Bergisch Gladbach, Germany) and anti-CD45-APC (diluted 1:5, BD Biosciences, Heidelberg, Germany) for another 15 min. Samples were washed again, fixed with 1% formaldehyde in PBS and analysed by flow cytometry. A gating strategy to exclude debris, doublets and high CD45 + cells was performed. Remaining GFP + /EpCAM + cells were analysed using version 4.07 of the FCS Express software (De Novo Software, Glendale, USA). Cell lines HEK-293 (ATCC CRL-1573), SK-OV-3 (ATCC HTB-77), MDA-MB-453 (ATCC HTB-131), CHO-K1 (ATCC CCL-61) and LNT-229 (ATCC CRL-2611) cells were grown in DMEM supplemented with 10% FCS and 1% glutamine. CHO-Her-k6 cells were cultivated in DMEM supplemented with 10% FCS and 1% glutamine and 1.2 mg ml −1 G418 (Invitrogen, Karlsruhe, Germany) [43] . A3.01 (ATCC CRL-2570), A2.01 (ATCC CCL-120.1), Raji (ATCC CCL-86) and Jurkat (ATCC TIB-152) cells were grown in RPMI medium supplemented with 10% FCS and 1% glutamine. For the generation of CHO-EpCAM cells, the cDNA sequence of human EpCAM (pCMV6-AC-EpCAMcDNA, Origene, Rockville, USA) and a puromycin resistance gene were cloned into a lentiviral transfer vector resulting in the bicistronic plasmid pS-hEpCAM-IRES-puro-W. CHO-K1 cells were transduced with lentiviral vector particles having packaged the hEpCAM-IRES-puro sequence and were selected using puromycin for 2 weeks. The resulting CHO-EpCAM bulk cell population was stained for EpCAM expression and a single clone named CHO-EpCAM H1 was selected for further experiments. For the generation of MDA-MB-453-luc cells, MDA-MB-453 cells were transduced with lentiviral vectors transferring the luciferase gene [44] at a multiplicity of infection of 0.5. A single-cell clone was analysed for luciferase and Her2/neu expression and was used for in vivo experiments. Statistics Data were analysed using the unpaired two-tailed t -test or repeated-measures analysis of variance. Survival curves were analysed by the Kaplan–Meier logrank test. P ≤0.05 was taken to be significant. Graph Pad Prism 5 provided the software for statistical analysis. How to cite this article: Münch, R. C. et al . Off-target-free gene delivery by affinity-purified receptor-targeted viral vectors. Nat. Commun. 6:6246 doi: 10.1038/ncomms7246 (2015).